Imaging neural spiking in brain tissue using FRET-opsin protein voltage sensors Genetically encoded fluorescence voltage sensors offer the possibility of directly visualizing neural spiking dynamics in cells targeted by their genetic class or connectivity. Sensors of this class have generally suffered performance-limiting tradeoffs between modest brightness, sluggish kinetics and limited signalling dynamic range in response to action potentials. Here we describe sensors that use fluorescence resonance energy transfer (FRET) to combine the rapid kinetics and substantial voltage-dependence of rhodopsin family voltage-sensing domains with the brightness of genetically engineered protein fluorophores. These FRET-opsin sensors significantly improve upon the spike detection fidelity offered by the genetically encoded voltage sensor, Arclight, while offering faster kinetics and higher brightness. Using FRET-opsin sensors we imaged neural spiking and sub-threshold membrane voltage dynamics in cultured neurons and in pyramidal cells within neocortical tissue slices. In live mice, rates and optical waveforms of cerebellar Purkinje neurons’ dendritic voltage transients matched expectations for these cells’ dendritic spikes. Optical microscopy using fluorescent protein voltage indicators is a promising, emerging method to monitor neural activity across ensembles of individual neurons identified by genetic or connectivity attributes [1] , [2] . Unlike small-molecule voltage sensors [3] , [4] , [5] , [6] , [7] , or hybrid approaches that combine genetically encoded fluorescent proteins with exogenous organic molecules [8] , [9] , voltage sensors that can be fully encoded genetically are readily amenable to combination with the substantial existing sets of genetic tools and viral delivery methods that enable long-term expression and chronic imaging experiments without addition of exogenous agents. To this point, genetically encoded fluorescent Ca 2+ indicators offer similar targeting advantages and have already had major impact on neuroscience research [10] . However, Ca 2+ imaging fails to reveal individual action potentials in many fast-spiking cell types, poorly captures sub-threshold membrane voltage dynamics and offers insufficient temporal information to permit studies of action potential timing to better than ~50–100 ms. Genetically encoded voltage indicators directly sense the transmembrane voltage and thus offer the possibility of faithfully observing action potential waveforms and sub-threshold voltage dynamics. One class of genetically encoded voltage sensors employs the Ciona intestinalis voltage-sensitive domain (Ci-VSD), which exhibits a voltage-dependent conformational change [2] . Combining Ci-VSD with pairs of bright fluorescent proteins that permit FRET yielded sensors that convert the voltage-dependent conformational alterations to changes in FRET efficiency and fluorescence intensities with response times of ~20–100 ms (ref. 2 ). Further engineering of the VSD, combined with brighter fluorophores of various colours, led to second-generation FRET voltage sensors (VSFP2.x, VSFP-mUKG-mKOκ, and VSFP-clover-mRuby variants) with superior voltage sensitivity [11] , [12] , [13] , [14] , [15] , [16] . Additional changes to both the VSD and fluorophore portions produced still further enhancements in dynamic range and kinetics [17] , [18] , [19] , [20] , [21] . Nevertheless, though Ci-VSD sensors have attained very high brightness due to their fluorescent protein components, they still exhibit limited dynamic response to action potentials (Δ F/F <3%), due to either weak voltage sensitivity or rise-time kinetics too slow to respond well to neural spikes. Notably, the sluggish kinetics of some sensors of this family, such as the VSFP3 variant Arclight [17] , [22] , preclude detailed studies of fast-spiking cell types or quantification of sub-threshold events—key raisons d’être for voltage sensor development. As an alternative to the combination of VSDs with fluorescent proteins, another class of protein voltage sensors has used rhodopsin family proteins traditionally employed for optically silencing neurons [23] . Spectroscopic studies of the proton pumping photocycle in bacteriorhodopsin and Archaerhodopsin (Arch) have revealed that proton translocation through the retinal Schiff base changes chromophore absorption [24] , [25] , [26] . Changes to the local electronic environment, such as by manipulating pH or trans-membrane voltage, likewise modulated the absorption spectrum of both proteorhodopsin and Arch [26] , [27] , and this effect conferred a voltage sensitivity to rhodopsin fluorescence. However, point mutations to Arch (for example, D95N) that eliminated the protein’s proton current also slowed both the photocycle and the sensor kinetics [26] . Recently, we reported mutations, Arch-EEN and Arch-EEQ, that sped the voltage-sensing kinetics and improved the dynamic range (Δ F/F >10% for action potentials), while maintaining negligible photocurrent [28] . The large dynamic range and fast kinetics enabled robust detection of action potentials in cultured neurons. Still, the main hindrance precluding the use of rhodopsin family sensors in brain slice or live animal preparations was the dim fluorescence, easily overwhelmed by tissue auto-fluorescence. To address the challenge of sensing voltage with sufficiently bright and rapid optical sensors, here we introduce FRET-opsin fluorescent voltage sensors that combine bright fluorescent proteins with the L. maculans (Mac) rhodopsin’s fast kinetics. This combination successfully reports fast trains of neural action potentials in cultured cells with substantial responses to action potentials (Δ F/F ≥5%), along with fourfold faster kinetics and a two- to fourfold increase in brightness compared with Arclight. We first describe the basic FRET-opsin design along with mutations that permit voltage sensing without light-driven photocurrent. By using signal detection theory to analyse our measurements, we find that FRET-opsin sensors report neural spikes with double the detection fidelity of Arclight, and thus exponentially reduced error rates for spike detection [29] . Lastly, we demonstrate use of FRET-opsin sensors to detect action potentials in neurons cultured in vitro and in neocortical pyramidal cells in brain tissue slices. In live mice, we detected voltage transients in the dendritic arbors of cerebellar Purkinje neurons, at rates and with optical waveforms that quantitatively fit expectations for the dendritic Ca 2+ spikes these cells exhibit. All of these studies used far lower illumination powers than originally required with Arch sensors [27] , [28] . Design of the FRET-opsin fluorescent voltage sensors The FRET-opsin sensors we constructed are fusions of a bright fluorophore, which acts as the FRET donor, to the Mac rhodopsin molecule, which serves as both the VSD and the FRET acceptor ( Fig. 1a , top). This approach was inspired by preliminary work using the FRET-opsin design with Arch [30] and prior work showing that bright fluorescent proteins bound closely to rhodopsin molecules can report changes in the rhodopsin absorption spectrum via FRET [31] . Mac has a slower photocycle and a blue-shifted action spectrum compared with Arch and NpHR [23] , [32] . We surmised that the slower photocycle might confer Mac with superior voltage sensitivity, as the slower states in the Arch photocycle are implicated in voltage sensitivity [33] . The blue-shifted action spectrum permits Mac’s use as a FRET acceptor in combination with a diverse set of fluorescent proteins, including blue, green and yellow fluorescent proteins. Notably, yellow fluorescent proteins derived from A. victoria are extremely bright fluorescent proteins and generally show minimal aggregation in live animal preparations. 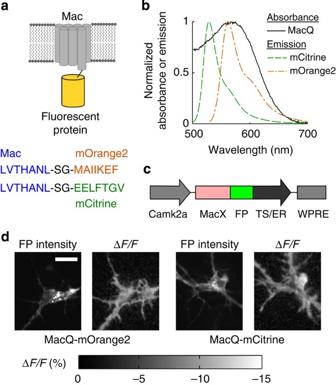Figure 1: Design and membrane localization of FRET-opsin sensor constructs in cultured neurons. (a) Top, cartoon of the Mac-fluorescent protein fusion. Bottom, amino-acid sequences of the linker for the Mac-mOrange and Mac-mCitrine sensors. (b) Emission spectra of the donor mCitrine and mOrange fluorescent proteins and the absorption spectrum of MacQ, the FRET acceptor. (c) We expressed the enhanced Mac constructs as a protein fusion with mOrange2/mCitrine under the control of theCamk2apromoter and targeted the fusion protein to the cell membrane using the localization sequences TS and ER. (d) Fluorescence signals from neurons labelled with MacQ-mOrange2 and MacQ-mCitrine. The left images of each set are from the fluorescent protein’s colour channel; the right images are spatial maps of the fluorescence response to a voltage step depolarization of ~100 mV. Regions of fluorescence and voltage response are generally colocalized. Scale bar is 20 μm and applies to all four images. Figure 1: Design and membrane localization of FRET-opsin sensor constructs in cultured neurons. ( a ) Top, cartoon of the Mac-fluorescent protein fusion. Bottom, amino-acid sequences of the linker for the Mac-mOrange and Mac-mCitrine sensors. ( b ) Emission spectra of the donor mCitrine and mOrange fluorescent proteins and the absorption spectrum of MacQ, the FRET acceptor. ( c ) We expressed the enhanced Mac constructs as a protein fusion with mOrange2/mCitrine under the control of the Camk2a promoter and targeted the fusion protein to the cell membrane using the localization sequences TS and ER. ( d ) Fluorescence signals from neurons labelled with MacQ-mOrange2 and MacQ-mCitrine. The left images of each set are from the fluorescent protein’s colour channel; the right images are spatial maps of the fluorescence response to a voltage step depolarization of ~100 mV. Regions of fluorescence and voltage response are generally colocalized. Scale bar is 20 μm and applies to all four images. Full size image We drew on the extensive literature regarding how protein mutations affect the bacteriorhodopsin photocycle, as well as our own prior work in Arch [28] , to convert Mac to a voltage-sensing domain. From the sequence homology between bacteriorhodopsin and Mac, we noted that proton pumping involves the two key amino acids, D139 and D150 (refs 34 , 35 , 36 ). Deprotonation of the Schiff base and donation of charge to the D139 residue is the first proton translocation step of the photocycle. Re-protonation of the Schiff base, with charge donated from the D150 position, is the final step [24] , [25] . Mutations at these key positions alter the dynamic range, photocurrent, and kinetics of voltage sensitivity in rhodopsin molecules [26] , [27] , [28] . We recapitulated the homologous mutations from our Arch studies [28] into Mac. First, we mutated D139 to an uncharged amino acid, which is a general way to eliminate photocurrent [26] , [28] , [34] , [35] , [36] . We employed the mutations D139N and D139Q, both of which dramatically slowed the photocycle and increased dynamic range when applied to the homologous positions in Arch [26] , [28] . The position homologous to D150 in Arch is the primary proton donor to the Schiff base that supports Arch’s voltage sensitivity. When combined with mutations homologous to D139N and D139Q, the homologous D150E mutation in Arch sped the kinetics by three- to ‘five-fold’ for parallel construction [28] . The resulting Arch sensors had rise-time constants of 5–15 ms and detected action potentials with Δ F/F >10% (ref. 28 ). We then screened the voltage sensitivity of Mac D139N (MacN), D139Q (MacQ), Mac D139N-D150E (Mac-EEN) and Mac D139Q-D150E (Mac-EEQ) using 633 nm illumination and detection of near-infrared emission (Methods). To our surprise, the D150E mutation slowed the kinetics of voltage-sensing; Mac-EEN and Mac-EEQ both had substantially longer decay times than MacN and MacQ, respectively ( Supplementary Fig. 1 ). However, MacN and MacQ had kinetic speeds comparable to Arch-EEN and Arch-EEQ (5–10 ms rise times), suggesting they might detect spikes well. We found that Mac fluorescence is even dimmer than Arch fluorescence, implying Mac cannot serve as an effective fluorescence sensor on its own. Thus, to create voltage sensors with dynamic range comparable to that of the Mac VSD but superior in brightness, we chose fluorescent proteins that can interact well with Mac via FRET in a fusion configuration ( Fig. 1a , top). Namely, such fluorescent proteins should have a high quantum yield and emission spectra that overlap substantially with Mac’s absorption spectrum. Wild-type Mac’s action spectrum peaks at 550 nm (ref. 23 ), so we chose mOrange2 and mCitrine as candidate FRET donors ( Fig. 1b ). To minimize the spatial separation between Mac and the donor protein, we chose what seemed to be the shortest workable linker between the two chromophores. Using crystal structures from bacteriorhodopsin as a template for Mac, and the crystal structures of mOrange2 and mCitrine, we trimmed Mac’s excess C terminus tail and the fluorescent proteins’ excess N terminus tails. This yielded the linker sequences for Mac-mOrange2 and Mac-mCitrine ( Fig. 1a , bottom); further reduction of the linker would very likely impair folding and localization to the cell membrane. We then employed the same trafficking motifs used previously with a broad class of inhibitory opsins [32] , [37] , [38] . The endoplasmic reticulum (ER) export sequence (FCYENEV) and the Golgi export trafficking signal (TS) sequence (KSRITSEGEYIPLDQIDINV), found in membrane-localized Kir2.1 potassium channels [39] , enhanced rhodopsin localization to mammalian neural membranes. These trafficking signals have previously improved both the photocurrent of rhodopsin ion pumps [32] , [37] , [38] and the signal-to-noise ratio (SNR) of Arch voltage sensors [28] . To minimize the distance between the two chromophores, we placed the trafficking signal at the end of the fusion construct ( Fig. 1c ), despite that it was previously placed between the opsin and fluorescent protein [32] , [38] . For studies in cultured neurons and brain slices, we generated FRET-opsin constructs containing a CaMKIIα (Camk2a) promoter and the woodchuck hepatitis post-transcriptional regulatory element (WPRE) ( Fig. 1c ). The terminal placement of the trafficking signals did not appear to adversely impact membrane localization, as fluorescence emission from the FRET donor channel was generally membrane-localized and revealed minimal intracellular aggregation in transfected neurons ( Fig. 1d , left panel of each pair). Moreover, image pixels that showed the greatest Δ F/F changes in response to a voltage step protocol were also membrane-localized, and colocalized with the baseline fluorescence signals ( Fig. 1d , right panel of each pair). This finding of membrane localization permitted us in subsequent characterizations to employ binned image pixels (3 μm × 3 μm) and therefore fast image acquisition rates (>400 Hz frame rates), because we did not have to computationally remove fluorescence contributions from mistargeted fluorescence aggregates in the cytosol (Methods). Such coarse-grained analyses allowed imaging studies over broad specimen areas while preserving the dynamic range of Δ F/F values. As wild-type inhibitory opsins generate photocurrent when illuminated with visible light, we characterized how the new mutants responded to illumination and energy transfer from the FRET donors. First using wild-type Arch for a reference measurement, we measured >300 pA photocurrent during visible illumination representative of that used during imaging ( λ =530 nm; 15 mW mm –2 at the specimen plane). Under the same illumination conditions as used throughout for MacQ-mOrange ( λ =530 nm; 15 mW mm –2 ) and MacQ-mCitrine ( λ =505 nm; 15 mW mm –2 ), MacQ displayed a transient excitatory photocurrent at illumination onset (–24±3 pA for 530 nm and –25±3 pA for 505 nm; mean±s.e.m. ; n =14 and 9 cells, respectively), and MacN displayed the same initial transient (–47±3 pA; mean±s.e.m. ; n =13; λ =530 nm) ( Fig. 2a,b ). During steady-state illumination, MacQ had negligible photocurrent (0.1±0.1 pA for 530 nm and –0.2±0.2 pA for 505 nm, mean±s.e.m. ; n =14 and 9 cells, respectively), unlike MacN, which exhibited sufficient steady-state photocurrent (–2.0±0.3 pA, λ =530 nm, mean±s.e.m. ; n =13 cells) to perturb neuron spiking patterns ( Supplementary Fig. 2 ). Thus, we used MacQ as the VSD for all subsequent experiments. 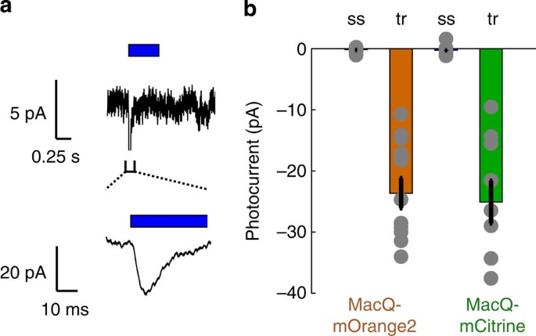Figure 2: MacQ-based sensors exhibit transient but not steady-state photocurrents. (a) MacQ constructs generate a transient excitatory photocurrent at the onset of illumination, illustrated here by the inward current (top) evoked by illumination (blue bars) of a neuron expressing MacQ-mOrange2. The steady-state photocurrent deviates negligibly from the baseline measured in the absence of illumination. An expanded view of the photocurrent transient (bottom) reveals its time course at the onset of illumination. (b) Steady-state (ss) and transient (tr) photocurrents of MacQ-mOrange2 (n=14 cells) and MacQ-mCitrine (n=9 cells) in response to 530 nm and 505 nm illumination, respectively. Illumination intensity at the specimen was 15 mW mm–2for all panels. Error bars are s.e.m. Figure 2: MacQ-based sensors exhibit transient but not steady-state photocurrents. ( a ) MacQ constructs generate a transient excitatory photocurrent at the onset of illumination, illustrated here by the inward current (top) evoked by illumination (blue bars) of a neuron expressing MacQ-mOrange2. The steady-state photocurrent deviates negligibly from the baseline measured in the absence of illumination. An expanded view of the photocurrent transient (bottom) reveals its time course at the onset of illumination. ( b ) Steady-state (ss) and transient (tr) photocurrents of MacQ-mOrange2 ( n =14 cells) and MacQ-mCitrine ( n =9 cells) in response to 530 nm and 505 nm illumination, respectively. Illumination intensity at the specimen was 15 mW mm –2 for all panels. Error bars are s.e.m. Full size image Characterization of FRET-opsin sensors in cultured neurons First, we compared the step responses of MacQ-mOrange2 and MacQ-mCitrine in cultured neurons ( Figs 3a,b and 4a ). Both sensors rose to 1−1/ e of their full response amplitudes in ~5 ms. This speed is comparable to that of the fastest Arch-EEX mutations [28] , and notably faster than Arclight’s 20 ms rise time ( Fig. 4a and Supplementary Table 1 ). In particular, the fast on-component of the MacQ sensor ( τ +,fast ~3 ms) was approximately fourfold faster than the fast on-component of Arclight ( τ +,fast ~12 ms). The steady-state Δ F/F responses of both MacQ sensors to applied voltage (~20% Δ F/F per 100 mV, computed from linear fits of the Δ F/F versus voltage relationships around the –70 mV holding potential; Fig. 3b ) underperformed Arclight-239Q (~35% Δ F/F per 100 mV), the Arclight variant of greatest voltage sensitivity. However, after taking into account their superior brightness, the two MacQ FRET-opsin sensors had steady-state SNR values comparable to or better than Arclight’s (Methods, Supplementary Fig. 3 ). We modelled the probes’ frequency responses, again taking SNR into account; the combination of faster kinetics and higher brightness led to superior responses for the Mac sensors at nearly all frequencies ( Fig. 4b ). The limited frequency response of Arclight was especially apparent during fast trains of spikes elicited by constant current injection ( Fig. 4c ). Owing to the substantial slow component of Arclight’s response to a sustained depolarization (~90 ms time constant accounting for ~40% of the full steady-state response; Supplementary Table 1 ), constant current injection led to prolonged increase in optical signal that made it challenging to separate spikes from sub-threshold membrane voltage dynamics ( Fig. 4c ). 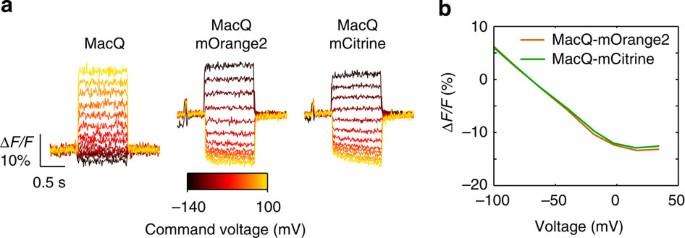Figure 3: FRET-opsin sensors report voltage depolarization via decreases in emission intensity from the fluorescence donor. (a) Optical step responses of cultured HEK293T cells transfected with MacQ, and cultured neurons transfected with MacQ-mOrange2 and MacQ-mCitrine (440 Hz frame rate). The MacQ VSD increased its fluorescence intensity with increased voltage depolarization (left). The donor fluorescent proteins of the FRET-opsin sensors exhibited decreases in fluorescence intensity with increased depolarization (middle, right). We held neurons at −70 mV at the start of each trace and stepped to command voltages ranging from −140 mV to +100 mV. (b) Steady state fluorescence responses of MacQ-mOrange2 and MacQ-mCitrine as a function of neuronal membrane voltage. Illumination at the specimen plane was 1,400 mW mm−2(λ=633 nm) for the MacQ studies, and 15 mW mm−2(λ=530 nm and 505 nm, for MacQ-mOrange and MacQ-mCitrine, respectively) for the FRET-opsin sensors. Error bars are s.e.m. Figure 3: FRET-opsin sensors report voltage depolarization via decreases in emission intensity from the fluorescence donor. ( a ) Optical step responses of cultured HEK293T cells transfected with MacQ, and cultured neurons transfected with MacQ-mOrange2 and MacQ-mCitrine (440 Hz frame rate). The MacQ VSD increased its fluorescence intensity with increased voltage depolarization (left). The donor fluorescent proteins of the FRET-opsin sensors exhibited decreases in fluorescence intensity with increased depolarization (middle, right). We held neurons at −70 mV at the start of each trace and stepped to command voltages ranging from −140 mV to +100 mV. ( b ) Steady state fluorescence responses of MacQ-mOrange2 and MacQ-mCitrine as a function of neuronal membrane voltage. Illumination at the specimen plane was 1,400 mW mm −2 (λ=633 nm) for the MacQ studies, and 15 mW mm −2 ( λ =530 nm and 505 nm, for MacQ-mOrange and MacQ-mCitrine, respectively) for the FRET-opsin sensors. Error bars are s.e.m. 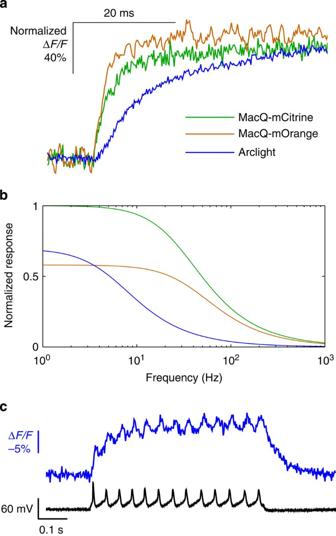Figure 4: The rapid kinetics of MacQ sensors provide a superior frequency response curve as compared with Arclight. (a) Step responses of the MacQ sensors and Arclight to command voltage steps of +100 mV from a holding of −70 mV, normalized to the maximum (or steady-state) ΔF/Fresponse to the command voltage (average ofn=3–6 trials for each construct). MacQ sensors exhibited three- to four-fold faster rise times than that of Arclight. Illumination intensities were 15–50 mW mm–2at the specimen plane. We used a photomultiplier tube to attain a 5 kHz data acquisition rate. (b) To estimate each voltage sensor’s frequency response curve, we used the step response measurements from (a), the sensors’ empirically determined brightness values, and the sensors’ empirically determined time constants (Methods). Our calculations assumed these time constants were invariant across different holding potentials and voltage steps. Although this assumption is surely wrong for large voltage changes, it simplified the calculations while providing basic insights. MacQ-mCitrine substantially outperformed Arclight at all frequencies, due to MacQ-mCitrine’s faster kinetics, higher brightness and superior SNR. (c) Electrophysiological and optical traces simultaneously acquired from a cultured neuron expressing Arclight (blue trace). The neuron exhibited repeated spiking during a period of constant current injection, and throughout the spike train there was a sustained increase in Arclight’s baseline fluorescence. As with isolated spikes, Arclight reported action potentials with small ΔF/F(<3%) values and without visible after-hyperpolarizations. Illumination intensity was 15 mW mm–2(λ=480 nm). The frame acquisition rate was 440 Hz. Full size image Figure 4: The rapid kinetics of MacQ sensors provide a superior frequency response curve as compared with Arclight. ( a ) Step responses of the MacQ sensors and Arclight to command voltage steps of +100 mV from a holding of −70 mV, normalized to the maximum (or steady-state) Δ F/F response to the command voltage (average of n =3–6 trials for each construct). MacQ sensors exhibited three- to four-fold faster rise times than that of Arclight. Illumination intensities were 15–50 mW mm –2 at the specimen plane. We used a photomultiplier tube to attain a 5 kHz data acquisition rate. ( b ) To estimate each voltage sensor’s frequency response curve, we used the step response measurements from ( a ), the sensors’ empirically determined brightness values, and the sensors’ empirically determined time constants (Methods). Our calculations assumed these time constants were invariant across different holding potentials and voltage steps. Although this assumption is surely wrong for large voltage changes, it simplified the calculations while providing basic insights. MacQ-mCitrine substantially outperformed Arclight at all frequencies, due to MacQ-mCitrine’s faster kinetics, higher brightness and superior SNR. ( c ) Electrophysiological and optical traces simultaneously acquired from a cultured neuron expressing Arclight (blue trace). The neuron exhibited repeated spiking during a period of constant current injection, and throughout the spike train there was a sustained increase in Arclight’s baseline fluorescence. As with isolated spikes, Arclight reported action potentials with small Δ F/F (<3%) values and without visible after-hyperpolarizations. Illumination intensity was 15 mW mm –2 ( λ =480 nm). The frame acquisition rate was 440 Hz. Full size image By comparison, the faster kinetics of the Mac sensors enabled detection of action potentials with high temporal accuracy and within fast trains of spikes ( Fig. 5a,b ). Typical optical traces (440 Hz frame-acquisition rate) corresponded well to simultaneously recorded traces of electrical activity, regarding both spiking and sub-threshold dynamics ( Fig. 5a–c ). We also determined the MacQ sensors’ peak Δ F/F values and optical waveforms in individual neurons for single action potentials induced by short current injections, and we compared these to the responses of the Arclight sensor ( Fig. 5c ). Electrophysiological recordings for cells expressing MacQ-mOrange2, MacQ-mCitrine and Arclight respectively revealed action potentials with durations (FWHM) of 2.9±0.8 ms, 3.2±0.6 ms and 3.3±0.9 ms (mean±s.d. ; n =10–12 cells), which are typical values for cultured neurons. Owing to its faster kinetics, MacQ sensors exhibited enhanced peak Δ F/F responses to neural spikes as compared with Arclight-239Q. MacQ-mOrange2 and MacQ-mCitrine had peak Δ F/F responses of 7.2±0.4% (mean±s.e.m. ; n =17 cells) and 4.8±0.2% (mean±s.e.m. ; n =12 cells), respectively. These values represent ~2.3-fold and ~1.6-fold increases over Arclight, respectively. 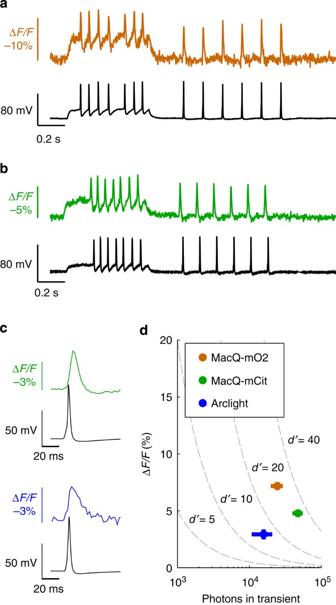Figure 5: Mac voltage sensors report single action potentials with higher spike detection fidelity than Arclight. (a,b) Optical traces from cultured neurons expressing (a) MacQ-mOrange2 (orange trace) and (b) MacQ-mCitrine (green trace) had sharp peaks that matched the action potentials in the simultaneously acquired electrophysiological traces (black). (c) Optical waveforms of single action potentials from MacQ-mCitrine (green trace, averaged overn=16 spikes) and Arclight (blue trace, average overn=10 spikes). The MacQ sensor has faster decay kinetics and reports the after-hyperpolarization phase of the spike waveform. (d) Peak ΔF/Fvalues of the optical responses to action potentials, plotted as a function of the total number of photons detected per spike. We estimated ordinate and abscissa values from the optical waveforms in panelc. Dashed lines are iso-contours of the spike detection fidelity,d′, which is determined by the sensor’s brightness, peak ΔF/Fand optical waveform29. Fluorescence imaging rates were 440 Hz for all panels, and the illumination intensity was 15 mW mm–2at the specimen plane for all sensors. Error bars are s.e.m. Figure 5: Mac voltage sensors report single action potentials with higher spike detection fidelity than Arclight. ( a,b ) Optical traces from cultured neurons expressing ( a ) MacQ-mOrange2 (orange trace) and ( b ) MacQ-mCitrine (green trace) had sharp peaks that matched the action potentials in the simultaneously acquired electrophysiological traces (black). ( c ) Optical waveforms of single action potentials from MacQ-mCitrine (green trace, averaged over n =16 spikes) and Arclight (blue trace, average over n =10 spikes). The MacQ sensor has faster decay kinetics and reports the after-hyperpolarization phase of the spike waveform. ( d ) Peak Δ F/F values of the optical responses to action potentials, plotted as a function of the total number of photons detected per spike. We estimated ordinate and abscissa values from the optical waveforms in panel c . Dashed lines are iso-contours of the spike detection fidelity, d′ , which is determined by the sensor’s brightness, peak Δ F/F and optical waveform [29] . Fluorescence imaging rates were 440 Hz for all panels, and the illumination intensity was 15 mW mm –2 at the specimen plane for all sensors. Error bars are s.e.m. Full size image FRET-opsin sensors have superior spike detection fidelity As described in prior work [29] , a sensor’s Δ F/F response and its brightness are both important contributors to the capabilities for spike detection. We characterized the MacQ sensors using metrics of SNR and spike detection fidelity and observed that the sensors substantially outperformed Arclight. A simplistic notion of SNR is the peak response divided by the s.d. of the baseline fluorescence in one time bin (Methods). We compared the shot-noise limited performance of the various sensors using this metric, under uniform imaging conditions (440 Hz frame rate; 15 mW mm –2 illumination) ( Supplementary Fig. 4 ). Bolstered by the two- to four-fold increase in brightness and four-fold increase in speed, MacQ-mOrange2 and MacQ-mCitrine respectively outperformed Arclight by 3.8-fold and 4.4-fold in this metric. We also used a signal detection theoretic framework to quantify the fidelity of spike detection [29] . The spike discriminability metric described in ref. 29 , denoted here as d′ , indexes the receiver-operating characteristic curve for spike detection and quantifies the degree to which spikes can be correctly identified within fluorescence data attained at the physical noise limits set by photon shot noise (Methods). This figure of merit takes into consideration a neuron’s experimentally determined fluorescence baseline, the peak Δ F/F response to a spike, and the temporal duration of the sensor’s response to a spike. By aggregating photons over multiple frames and accounting for sensor kinetics, this framework provides a far more realistic measure of spike detection fidelity than more traditional, simplistic measures of SNR such as that shown in Supplementary Fig. 4 . To compare spike discriminability, we combined onto one plot the iso-contours of d′ , the sensors’ peak Δ F/F values and the total number of photons aggregated within a fluorescent transient, all obtained from our experimental determinations of peak Δ F/F values and the photon shot noise in the baseline fluorescence emissions ( Fig. 5d , Methods). The slow kinetics of Arclight yielded longer transients that provided partial compensation for its inferior peak Δ F/F value compared with the Mac sensors. However, MacQ-mOrange2 and MacQ-mCitrine still outperformed Arclight, by factors of 1.8 and 2.2 in d ′, respectively. In the framework of the receiver-operating characteristic, a doubling of d’ sharply reduces errors in spike detection since it yields far more than a squaring of the detection error probability [29] . The d′ values determined here predict that Mac sensors should theoretically exhibit a ~10 8 -fold reduction in spike detection error rates as compared with Arclight. Such a huge improvement is unattainable under true experimental conditions, due to noise sources other than photon shot noise, but this calculation illustrates the large impact of even modest increases in spike detection fidelity. Although d ′ is a measure of detection fidelity for temporally isolated spikes, sensors such as MacQ with faster kinetics also enable discrimination of individual spikes within rapid spike bursts. MacQ-mCitrine enables spike detection in live brain slices We next examined the ability of the MacQ sensors to sense voltage in a variety of slice and in vivo preparations. We used in utero electroporation to deliver the sensors to the neocortex [21] , and observed bright expression for both sensors ( Fig. 6a ). As is often typical of fusions of rhodopsins with fluorescent proteins derived from the Anthozoa red fluorescent protein [40] , the MacQ-mOrange2 sensor showed significant intracellular aggregation ( Fig. 6a , right). On the other hand, fusions of rhodopsins with fluorescent proteins derived from A. Victoria generally do not show aggregations [32] , [37] , [40] , and the MacQ-mCitrine fusion also showed desirable levels of membrane targeting ( Fig. 6a , left). Consequently, for all subsequent brain slice and in vivo studies, we used the MacQ-mCitrine sensor. 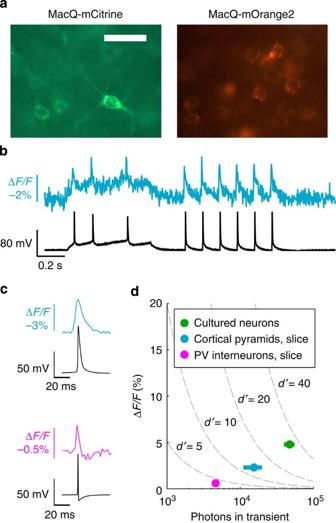Figure 6: MacQ-mCitrine reports spikes from excitatory neurons in brain slices. (a) Fluorescence images of neocortical neurons in fixed brain tissue from mice electroporatedin uterowith Mac sensors. Neurons electroporated with MacQ-mCitrine (left) exhibited minimal protein aggregation, whereas neurons electroporated with MacQ-mOrange2 (right) showed substantial aggregation. Scale bar, 20 μm. (b) In a brain slice recording followingin uteroelectroporation, MacQ-mCitrine fluorescence (cyan trace) from a layer 2/3 cortical pyramidal neuron matches the cell’s simultaneously recorded electrophysiological trace (black). (c) Optical waveforms for single action potentials from MacQ-mCitrine targeted to layer 2/3 neocortical pyramidal neurons (top, averaged overn=10 spikes) or from hippocampal parvalbumin interneurons (bottom, averaged overn=60 spikes) correspond well to the simultaneously recorded electrophysiological waveforms. (d) Peak ΔF/Fvalues of the optical responses to action potentials, as a function of the total number of photons detected per spike. We measured the values of peak ΔF/Fin live neocortical slices with MacQ-mCitrine in pyramidal neurons or parvalbumin (PV) interneurons, and estimated the abscissa values from the optical waveforms of panelc. The data from studies in cultured neurons are shown for reference. Dashed lines are iso-contours of spike detection fidelity,d′.Fluorescence imaging rates were 440 Hz for all panels; illumination intensity was 30 mW mm–2for all sensors. Error bars are s.e.m. Figure 6: MacQ-mCitrine reports spikes from excitatory neurons in brain slices. ( a ) Fluorescence images of neocortical neurons in fixed brain tissue from mice electroporated in utero with Mac sensors. Neurons electroporated with MacQ-mCitrine (left) exhibited minimal protein aggregation, whereas neurons electroporated with MacQ-mOrange2 (right) showed substantial aggregation. Scale bar, 20 μm. ( b ) In a brain slice recording following in utero electroporation, MacQ-mCitrine fluorescence (cyan trace) from a layer 2/3 cortical pyramidal neuron matches the cell’s simultaneously recorded electrophysiological trace (black). ( c ) Optical waveforms for single action potentials from MacQ-mCitrine targeted to layer 2/3 neocortical pyramidal neurons (top, averaged over n =10 spikes) or from hippocampal parvalbumin interneurons (bottom, averaged over n =60 spikes) correspond well to the simultaneously recorded electrophysiological waveforms. ( d ) Peak Δ F/F values of the optical responses to action potentials, as a function of the total number of photons detected per spike. We measured the values of peak Δ F/F in live neocortical slices with MacQ-mCitrine in pyramidal neurons or parvalbumin (PV) interneurons, and estimated the abscissa values from the optical waveforms of panel c . The data from studies in cultured neurons are shown for reference. Dashed lines are iso-contours of spike detection fidelity, d′. Fluorescence imaging rates were 440 Hz for all panels; illumination intensity was 30 mW mm –2 for all sensors. Error bars are s.e.m. Full size image First, we used the MacQ sensors to detect action potentials in excitatory cortical layer 2/3 neurons of the neocortex. Typical fluorescence traces tracked well the simultaneously recorded electrophysiological traces ( Fig. 6b ), and the fluorescence waveforms for action potentials matched their electrical counterparts ( Fig. 6c , top). As compared with cultured neurons, optical traces from cortical neurons in slice preparations suffered a decrease of ~50% in brightness and a decrease of ~50% in Δ F/F . We attributed the reduction in brightness to light scattering within the sliced tissue and a decrease in expression of the plasmid vector in vivo . We attributed the decrease in Δ F/F to increased background fluorescence, from both auto-fluorescence and out-of-plane fluorescence from labelled neuronal processes. As compared with cultured neurons, these differences resulted in declines of 70% in SNR and 60% in d′ ( Fig. 6d ). Nevertheless, the MacQ-mCitrine sensor enabled high-fidelity ( d′ >10) detection of single action potentials from single cortical neurons in slice preparations. There are possibilities for further improvements by upgrading the optical instrumentation. We also demonstrated genetic targeting of voltage sensors to specific neuron populations via the Cre-lox genetic targeting system. In particular, we created a double-floxed inversed open reading frame (DIO) construct with the CAG promoter, the MacQ-mCitrine insert and the WPRE after the insert ( Supplementary Fig. 5a ). This construct was intended to leverage the many available Cre mouse lines that express Cre-recombinase in selected cell types. The Cre-recombinase excises the lox sites from the sequence and orients the open reading frame such that the insert is transcribed under the control of the CAG promoter, thereby expressing the voltage sensor selectively in the chosen cell type. To illustrate, we used the Parv-IRES-Cre (Parv-Cre) mouse line, which expresses Cre-recombinase in parvalbulmin-positive neurons throughout the brain. We injected our AAV-CAG-DIO-MacQ-mCitrine construct into the hippocampus of Parv-Cre mice, and observed expression outside of the pyramidal neuron layer (sp) of the hippocampus, in the oriens-lacunosum moleculare interneurons of the stratum oriens (so) and the bistratified interneurons of the stratum radiatum (sr) ( Supplementary Fig. 5b ). We inferred that the labelled neurons were inhibitory interneurons during electrophysiological measurements, as the labelled neurons all had brief action potentials (FWHM<0.6 ms) ( Fig. 6c , bottom). In addition, we observed fast spiking without accommodation in these neurons ( Supplementary Fig. 5c ). However, we observed a large decrease in the peak responses to action potentials (Δ F/F =0.6%) as compared with the fluorescence transients seen in response to pyramidal neurons’ spikes ( Fig. 6c,d ). We attributed this sharp decline in dynamic range to the millisecond kinetics of the probe, which does not fully follow the sub-millisecond spike waveforms of fast-spiking interneurons. The probe attained a d′ value of ~4 when detecting interneuron spikes ( Fig. 6d ), considerably lower than the values attained for pyramidal spikes and near the threshold of accurate spike detection [29] . Nevertheless, MacQ-mCitrine had sufficiently fast kinetics to report aspects of high frequency oscillatory dynamics, such as that arising in interneurons during periodic spike trains of nearly ~100 Hz ( Supplementary Fig. 5c,d ). Optically detected voltage transients from Purkinje neurons To assess our capabilities for imaging individual neurons’ action potentials in live mice, we selected cerebellar Purkinje neurons for study ( Fig. 7a–e ). We reasoned that the dendritic Ca 2+ spikes these cells exhibit should provide among the most favourable conditions available for imaging individual action potentials in the live mammalian brain. Although the peak depolarization (+40−60 mV) in the dendrites is not as large as that for conventional (Na + ) spikes in neuronal cell bodies, the Ca 2+ spikes’ far longer durations (~5–10 ms, versus ~1–2 ms for Na + spikes) should more than compensate for the lesser depolarization and thereby generate a signal of greater detection fidelity than that of Na + spikes. Moreover, Purkinje neurons’ dendritic trees are highly elaborated and extend ~100–200 μm in the rostral–caudal dimension [41] , providing a far greater membrane surface area than a typical ~10 μm-diameter cell soma. Thus, although imaging of individual neuronal action potentials in the live mammalian brain had not been previously reported using genetically encoded voltage indicators, Purkinje neurons’ dendritic Ca 2+ spikes seemed to be a near-optimal action potential for our first attempt. 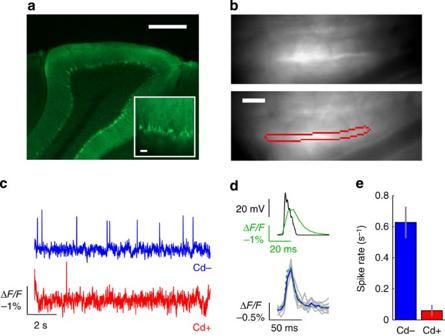Figure 7: The MacQ-mCitrine sensor reports voltage transients in the dendrites of Purkinje neurons in live mice. (a) Fluorescence image of MacQ-mCitrine expressed in cerebellar Purkinje neurons, as seen in a fixed tissue slice. Scale bar, 400 μm. Inset: magnified image of neurons expressing the voltage sensor reveals minimal sensor aggregation. Scale bar, 20 μm. (b) Epi-fluorescence image, acquired in an anaesthetized mouse, of Purkinje neurons’ dendritic trees expressing (top) MacQ-mCitrine, and with the region of interest (enclosed within the red perimeter) used to estimate the fluorescence trace for an individual Purkinje neuron dendritic tree (bottom). Scale bar, 40 μm. (c) Fluorescence traces averaged across the dendritic region of interest in panelbshowed transient depolarization events at rates consistent with those of dendritic Ca2+spikes in the cerebellar molecular layer44,45(blue trace). Application of the Ca2+channel inhibitor CdCl2largely abolished these events (red trace), as expected for Ca2+spikes46. Image acquisition rate was 190 Hz. Illumination intensity was 10 mW mm–2. (d) To estimate the expected optical waveform from a Purkinje neuron’s dendritic spike, we used as the basis for calculations the Ca2+spike’s voltage waveform as recorded electrically in the dendritic tree ~65 μm from the cell body42(top, black trace). By taking into account the kinetics and voltage-dependence of MacQ-mCitrine’s fluorescence emissions (Methods), we then computed the expected optical waveform of a single Ca2+spike (top, green trace). The experimentally determined optical waveforms from individual Purkinje neurons (bottom, grey traces) and their mean (bottom, blue trace) closely matched the theoretically predicted time course (bottom, dashed green trace). However, the calculated peak ΔF/Fresponse (1.7%) overestimated the peak of the average measured response (1.2%); we attribute the discrepancy to additional background photon emissions and noise fluctuations present in live mice that are absent in brain slices. (e) The mean detected rate of dendritic voltage transients before and after application of CdCl2(n=5 Purkinje neurons). Error bars are s.e.m. Figure 7: The MacQ-mCitrine sensor reports voltage transients in the dendrites of Purkinje neurons in live mice. ( a ) Fluorescence image of MacQ-mCitrine expressed in cerebellar Purkinje neurons, as seen in a fixed tissue slice. Scale bar, 400 μm. Inset: magnified image of neurons expressing the voltage sensor reveals minimal sensor aggregation. Scale bar, 20 μm. ( b ) Epi-fluorescence image, acquired in an anaesthetized mouse, of Purkinje neurons’ dendritic trees expressing (top) MacQ-mCitrine, and with the region of interest (enclosed within the red perimeter) used to estimate the fluorescence trace for an individual Purkinje neuron dendritic tree (bottom). Scale bar, 40 μm. ( c ) Fluorescence traces averaged across the dendritic region of interest in panel b showed transient depolarization events at rates consistent with those of dendritic Ca 2+ spikes in the cerebellar molecular layer [44] , [45] (blue trace). Application of the Ca 2+ channel inhibitor CdCl 2 largely abolished these events (red trace), as expected for Ca 2+ spikes [46] . Image acquisition rate was 190 Hz. Illumination intensity was 10 mW mm –2 . ( d ) To estimate the expected optical waveform from a Purkinje neuron’s dendritic spike, we used as the basis for calculations the Ca 2+ spike’s voltage waveform as recorded electrically in the dendritic tree ~65 μm from the cell body [42] (top, black trace). By taking into account the kinetics and voltage-dependence of MacQ-mCitrine’s fluorescence emissions (Methods), we then computed the expected optical waveform of a single Ca 2+ spike (top, green trace). The experimentally determined optical waveforms from individual Purkinje neurons (bottom, grey traces) and their mean (bottom, blue trace) closely matched the theoretically predicted time course (bottom, dashed green trace). However, the calculated peak Δ F/F response (1.7%) overestimated the peak of the average measured response (1.2%); we attribute the discrepancy to additional background photon emissions and noise fluctuations present in live mice that are absent in brain slices. ( e ) The mean detected rate of dendritic voltage transients before and after application of CdCl 2 ( n =5 Purkinje neurons). Error bars are s.e.m. Full size image To gauge our expectations, we first calculated the optical waveform expected from an individual Purkinje neuron’s dendritic spike. We approximated the dendritic spike’s voltage waveform as that recorded electrically in vitro in the dendritic tree ~65 μm from the cell body [42] ( Fig. 7d , top). Using the kinetics and voltage-dependence of MacQ-mCitrine’s fluorescence emissions (as in Fig. 4b ), we then computed the expected optical waveform of a single dendritic spike ( Fig. 7d , top). Owing to MacQ-mCitrine’s finite rise-time in response to a depolarization and the limitations imposed by our imaging frame rate, this computed waveform contained no indication of back-propagating Na + spikelets that can ride atop the Ca 2+ action potential of 5–10 ms duration in the Purkinje neuron dendrites [42] , [43] ( Fig. 7d ). Reflecting the sensor’s finite decay time, the expected optical waveform persisted for ~10 ms longer than the electrical transient. Having computed the expected signals, we injected an AAV-Camk2a-MacQ-mCitrine vector into the mouse cerebellar cortex to express the voltage reporter in Purkinje neurons ( Fig. 7a ). We then sought to detect voltage transients in these neurons’ dendritic arbors in live mice, using a cranial window preparation and epi-fluorescence microscopy (Methods). We chose focal planes within the cerebellar molecular layer, where Purkinje neurons’ dendritic trees lie, and imaged the transduced neurons ( Fig. 7b ) using similar imaging conditions as for our in vitro studies (10 mW mm –2 ). The resulting optical traces of voltage dynamics revealed that individual Purkinje neurons produced dendritic voltage transients at rates of 0.2–1 Hz, similar to the reported rates of dendritic spiking in mouse Purkinje neurons [44] , [45] ( Fig. 7e ), which are slightly lower than typical rates in other mammalian species. We then compared the optical waveforms for these voltage transients to the calculated expectations ( Fig. 7d , bottom). The shapes of the individual optical waveforms, and their mean, closely matched the time course of our computational prediction. However, the calculated peak Δ F/F response (1.7%) overestimated the peak of the average measured response (1.2%); we attribute the discrepancy to additional background photon emissions and noise fluctuations present in live mice that are absent in brain slices. Nevertheless, the shapes of the measured optical waveforms were a striking fit to that of the calculated optical response. We also attained simultaneous recordings from nearby Purkinje neurons ( Supplementary Fig. 6 ), suggesting the possibility of imaging populations of Purkinje neurons at the single-cell level with high temporal resolution. To further test the supposition that the voltage transients we measured optically were dendritic Ca 2+ spikes, we applied the Ca 2+ channel blocker CdCl 2 to the cerebellar cortex [46] . As expected for spikes based on Ca 2+ , this manipulation nearly completely abolished the voltage transients from the optical traces ( Fig. 7c,e ). Given the pharmacological rate and waveform evidence that the optically recorded voltage transients were consistent with those of dendritic Ca 2+ spikes, we sought definitive proof by attempting simultaneous optical and electrical recordings in the very same Purkinje neurons in live mice. Despite multiple attempts, the additional brain motion artifact incurred by making a small opening in the cranial window for insertion of the electrode was sufficient to obliterate the ~1% Δ F/F spiking signals attained prior to making the opening. Specifically, with a 0.13 mm 2 opening permitting a sideways insertion of the electrode, the additional brain motion caused a rise in the baseline fluorescence fluctuations, from 0.11% to 0.48% Δ F/F . This in turn lowered d′ from >10 to only ~2.5. Given our imaging rate (190 Hz), and the frequency of dendritic Ca 2+ spikes (~0.5 Hz), these numbers implied the lack of any spike detection threshold that could well separate actual spikes from false positives. For instance, even a high detection threshold that correctly captured only 50% of all dendritic Ca 2+ spikes still would have suffered fivefold more false-positive events than true positives. By comparison, before making the cranial window, d′ >10 implied mathematically the feasibility of setting a detection threshold attaining a total error rate of only ~10 −3 %. Overall, the evidence that the optical signals we saw represented dendritic Ca 2+ spikes came solely from the spike rate, Ca 2+ channel blockade, and waveform data, as we did not achieve satisfactory paired optical and electrical recordings. We constructed a Mac-based FRET-opsin voltage sensor that outperforms the previously published sensors by over a factor of 2 in d′ . This superior spike detection fidelity stems from the factors of ~4 × increase in speed, ~2–4 × increase in brightness and ~4 × increase in traditional SNR. We have demonstrated imaging experiments in cultured neurons and brain slice preparations in which we imaged the spiking patterns and membrane potential dynamics of single neurons of various genetically defined cell types. The high SNR of the MacQ-mCitrine probe overcame the substantial background and autofluorescence emissions present in one-photon epi-fluorescence imaging studies. Owing to the sharply nonlinear dependence of spike detection fidelity on d′ values, the increase of d′ by a factor of 2 should substantially improve the prospects of imaging voltage in more challenging preparations with low SNR. As a mathematical example, an improvement from d′ =2 to d′ =4 should decrease the spike detection error from ~10 −1 to ~10 −3 . Armed with these improvements in voltage sensing, we have described the first experiments to image the voltage dynamics of individual neurons in a live mammalian brain using a genetically encoded indicator. The rate and optical waveforms we observed for the dendritic spikes of cerebellar Purkinje neurons matched expectations based on the frequency and electrical time course of these events in the mouse cerebellar molecular layer. Cd 2+ abolished their occurrence, as expected for an action potential based on Ca 2+ . However, Cd 2+ blocks a wide range of Ca 2+ signalling pathways, including synaptic transmission, so this finding does not provide definitive proof that the events we saw were Ca 2+ spikes. Our attempts to attain superior evidence via dual optical and electrical recordings in live mice repeatedly failed, at core due to the limitations of the MacQ-mCitrine sensor. The peak ~1% Δ F/F spiking signals from the putative Ca 2+ spikes were insufficient to overcome the additional brain motion that occurred once we created a small opening in the cranial window to insert the electrode. This stands in marked contrast to the prior experiences of multiple laboratories, including our own, in performing simultaneous in vivo electrical and Ca 2+ imaging studies of individual Purkinje neurons’ dendritic spiking dynamics [47] , [48] , [49] . Ca 2+ indicators provide far superior optical signals (~20% Δ F/F ) for detection of Purkinje neurons’ dendritic Ca 2+ spikes, and the concordance between the electrically and optically recorded spike trains in these studies [47] , [48] , [49] is often >90%. For our voltage-imaging studies, given the evidence regarding the voltage transients’ Ca 2+ dependence, rate and waveforms, we conclude it is highly likely these transient were dendritic Ca 2+ spikes. However, this initial attempt at in vivo recording of single neuron dynamics in the live mammalian brain can only be seen as a partial success, at best. MacQ-mCitrine’s capabilities are notably superior to those of Arclight and prior genetically encoded voltage indicators, but the capacity to record neuronal action potentials in the live mammalian brain remains on the cusp of feasibility. Nevertheless, given that modest improvements in SNR and d′ values can have substantial benefits for spike detection fidelity, in vivo optical recordings of individual neurons’ voltage dynamics might be nearly at hand, at least for some cell types. The present capabilities of the FRET-opsin sensors introduced here indicate the substantial promise of this new class of voltage reporters, and we are optimistic about the prospects for future improvements. Regardless of its emission properties, Mac detects voltage transients with relatively large dynamic range and fast kinetics, and can serve as an adequate VSD. FRET-opsin sensors that combine rhodopsin VSDs with evolved fluorescent proteins offer a flexible design configuration, for which further development of the VSD can occur separately and in parallel with development of the fluorescence readout. This sensor design can incorporate enhancements in VSD kinetics and dynamic range, coming from mutations of existing proton-pumping rhodopsins or discovery of new rhodopsins, as well as new fluorescent proteins with increased brightness and photostability. A recent study done in parallel reports FRET-opsin sensors that use Archaerhodopsin as the FRET acceptor [50] . In contrast to the FRET-opsin sensors described here, ASAP1 (Accelerated Sensor of Action Potentials) is a newly reported voltage sensor formed by the insertion of a circularly permuted GFP into a chicken voltage-sensitive phosphatase [51] . Both sensor types have comparably fast kinetics, substantial responses to action potentials, and can report single neuronal spikes in live brain slices. Future studies that further elucidate the biophysical mechanisms of voltage-sensing in both rhodopsin family proteins and voltage-sensitive phosphatases are likely to promote additional improvements in sensor performance. Voltage sensors are likely to play different roles than Ca 2+ sensors in neuroscience research. The most recent genetically encoded Ca 2+ sensors are approaching reliable, single spike sensitivity, although their slow kinetics limits them to detecting temporally sparse action potentials [52] , [53] , such as those from neocortical pyramidal neurons. Genetically encoded voltage sensors will have important roles in detecting neural activity poorly captured by Ca 2+ sensors and quantifying key temporal aspects of neural dynamics. For example, although genetically encoded Ca 2+ sensors can resolve inter-spike intervals of <100 ms through multi-trial averaging [52] , voltage sensors such as the ones described here remain better candidates for imaging neural activity faster than 10 Hz in single-shot experiments. Unlike most Ca 2+ sensors, voltage sensors report sub-threshold dynamics as well as spiking dynamics. We have described here the first study of genetically targeted voltage imaging of interneurons, which will open the possibility of monitoring sub-threshold network oscillatory dynamics in both excitatory and inhibitory populations, phenomena that have largely been beyond Ca 2+ sensors’ capabilities. Further, Ca 2+ sensors report an ionic proxy of voltage dynamics, and thus have substantial variance in their fluorescence waveforms in response to single action potentials, as well as substantial variations in waveform across different cell types [52] , [53] . Voltage sensors respond to stereotyped action potentials with fixed, temporally precise waveforms that can avoid the saturation effects that impact Ca 2+ imaging. Thus, voltage imaging will also have a role in precisely quantifying neural activity, moving beyond binary detection of neural spikes by adding temporally precise descriptions of rate or temporal codes. However, as with Ca 2+ sensors, voltage indicators will have varying utility in different cell types, depending on the details of the action potential waveform, sub-threshold membrane dynamics, and the ability to keep background labelling to a minimum. MacQ-mCitrine reliably reports spiking dynamics of pyramidal neurons in brain slice preparations, but less so for fast-spiking (parvalbumin) interneurons ( Fig. 6c ). The latter cell type has brisker action potentials, and the FRET-opsin sensor does not track the spike waveform nearly as well as the longer lasting spikes that pyramidal cells emit. For all cell types, reduction of background labelling and photon emission is key, for unlike Ca 2+ sensors that are generally cytosolic, productive voltage sensor molecules are limited to the cell membrane. Thus, further improvements in both labelling methods and the voltage sensors themselves remain important pursuits for neuroscience research. Ethics statement The Stanford University Administrative Panel on Laboratory Animal Care (APLAC) approved all animal experiments. Sensor constructs Mac mutants originated from eMac3.0-GFP (Addgene plasmid 35515), in which the construct was expressed via the Camk2a promoter. We constructed all Mac variants by site-directed mutagenesis, and subsequent overlap assembly with mOrange2, mCitrine and trafficking signals. We made the pAAV-CAG-DIO Mac construct by inserting the MacQ-mCitrine construct into a pAAV-CAG-DIO backbone using the AscI and PstI restriction sites. The Mac variants are on Addgene as 48761 (MacQ-mOrange2) and 48762 (MacQ-mCitrine). For direct comparisons to the Mac constructs, we also placed Arclight 239Q under the control of the Camk2a promoter. Absorption and emission spectra We obtained MacQ’s absorption spectra by placing the rhodopsin under the cytomegalovirus (CMV) promoter and transfecting HEK cells at a total volume of 200 ml for 3 days. We added all-trans retinal (5 μM) and cultured the cells in the dark for 3 h. We pelleted the cells, lysed them using a sonicator in 50 mM Tris with 2 mM MgCl 2 at pH 7.3, and pelleted again. Finally, we homogenized the lysate in a solution (pH 7.2) containing 30 mM K 2 HPO 4 , 20 mM KH 2 PO 4 , 300 mM NaCl and 1.5% N -Octyl-β- D -Glucopyranoside (Sigma), and pelleted once more. We obtained the absorption spectrum using the supernatant and a spectrophotometer (Tecan Safire 2 UV–vis). Primary cell culture We dissected rat hippocampal cells from Sprague-Dawley pups (postnatal day 0, Charles-River Labs) and cultured them in Neurobasal media (Invitrogen), supplemented with glutamine and B27 (Invitrogen). We transfected Mac mutant plasmid DNA using calcium phosphate treatment 3–5 days after plating, and imaged the neurons 3–5 days after transfection. HEK293 cell culture We cultured HEK293T cells (Tribioscience, Palo Alto, CA, USA) in DMEM (Invitrogen) supplemented with glutamine (Invitrogen), fetal bovine serum (Invitrogen, 10% by vol), and streptomycin. We transfected Mac mutant plasmid DNA with Lipofectamine 2000 (Invitrogen) 1 day after plating, and imaged the cells 2 days after transfection. In utero electroporation Pregnant mice (CD-1; Jackson) underwent electroporation surgery under isoflurane (1.5–2%, vol/vol in O 2 ) at day E15.5. We removed embryos from the abdominal cavity and visualized them through the uterus. Using a glass capillary we injected 1 μl of Mac constructs at 1 μg μl –1 along with 0.05% fast green tracking dye (Sigma) into the lateral ventricle. We then applied five electric pulses (50 V, 50 ms) at 1 Hz to the neocortex with electrode forceps (Harvard Apparatus) connected to a square-pulse generator (Harvard Apparatus ECM 830). We obtained neocortical brain slices 3–5 weeks after birth. Adeno-associated virus production To create AAV gene delivery vectors, we employed and modified published procedures [54] , [55] . We purchased AAV expression, packaging and helper plasmids from the Penn Vector Core at University of Pennsylvania and transfected them into HEK293T cells (Tribioscience, Palo Alto, CA, USA) with calcium phosphate. We harvested the cells 3 days later, lysed them using the ADV/AAV release kit (Cell Lab Tech, Palo Alto, CA, USA), and centrifuged the solution to remove the cell debris. We purified the virus by loading the virus solution on iodixanol gradient media, followed by ultracentrifugation. We harvested 40% of the iodixanol layer, diluted it with phosphate-buffered saline (PBS), concentrated the virus and removed the iodixanol by using ultracentrifuge tube filters. We determined the viral titres by quantitative PCR using purified viral DNA (GeneAll, Korea). Virus injection For in vitro imaging studies of hippocampal tissue, we injected AAV2/5-CAG-DIO-MacQ-mCitrine (500 nl) into CA1 (–1.8 mm from Bregma, 1.4 mm mediolateral, –1.65 mm dorsoventral) of male Parv-IRES-Cre mice (12–16 weeks old). For in vivo imaging studies of cerebellum, we injected AAV2/1-Camk2a-MacQ-mCitrine into the cerebellum of wild-type male C57/bl6 mice aged 6–14 weeks (Lobule V, ±500 μm mediolateral, 200–700 μm anterior to Lobule VI, at a depth of 150–350 μm). In both cases, during the stereotactic injections mice received isoflurane anaesthesia (1.5–2%, vol/vol in O 2 ). Imaging experiments were 3–5 weeks after viral injection. Brain slices We dissected the intact mouse brain and placed the brain in electrolytic sucrose slicing solution containing 85 mM NaCl, 75 mM sucrose, 2.5 mM KCl, 25 mM glucose, 1.25 mM NaH 2 PO 4 , 4 mM MgCl 2 , 0.5 mM CaCl 2 and 24 mM NaHCO 3 , while bubbling carbogen (5% CO 2 , 95% O 2 ). We cut 300–350 μm thick slices using a vibratome (Leica VT1000S). Electrophysiology We simultaneously obtained fluorescence measurements and voltage or current clamp measurements at 22 °C while holding neurons in a perfusion chamber mounted on the microscope stage. The extracellular solution for cultured neurons contained 150 mM NaCl, 4 mM KCl, 10 mM glucose, 10 mM HEPES, 2 mM CaCl 2 and 2 mM MgCl 2 . The extracellular solution for slice experiments was ACSF, containing 3 mM KCl, 11 mM glucose, 123 mM NaCl, 1.25 mM NaH 2 PO 4 , 1 mM MgCl 2 and 2 mM CaCl 2 , and was bubbled with carbogen during the experiment. The intracellular solution contained 129 mM K-gluconate, 10 mM KCl, 10 mM HEPES and 4 mM Na 2 ATP. We pulled patch pipettes made of borosilicate glass to resistances of 3–6 MΩ (Sutter Instruments P-97), yielding access resistances of 5–25 MΩ in whole-cell mode. We patched neurons using an Axopatch 700B amplifier (Axon Instruments) and used pClamp software (Axon Instruments) to generate the various control waveforms and to record voltage and current traces. The voltage control waveform applied a holding potential of –70 mV at the start of each cycle and then applied steps lasting 1 s to voltages ranging from –140 mV to +100 mV in 20 mV increments. To generate action potentials in current clamp, we injected current using both long pulses (10–200 pA; >0.5 s) or short pulses (300–1,000 pA; 2 ms). The short current pulses triggered spikes with near unity efficiency when tuned above the spiking threshold, and with ~50% efficiency when near the spiking threshold. We made post hoc corrections to the membrane voltage measurements to account for the junction potential and access resistance. Fluorescence imaging We used an epi-fluorescence microscope (Olympus IX51) with a × 40 0.8 NA water immersion objective (LUMPlanFL 40XW, Olympus) for time-lapse imaging of cultured neurons and brain slices. We used a × 20 1.0 NA water immersion objective (XLUMPlanFL 20XW, Olympus) for imaging Purkinje neurons in vivo . For imaging MacQ-mCitrine in culture and slice preparations, we used a 505 nm LED (Thorlabs) for illumination, a 500/20 nm excitation filter, a 515 nm dichroic mirror and a 520 nm long-pass emission filter. For MacQ-mOrange2, we used the 530 nm LED from a Heliophore (89 North), a 530/30 nm excitation filter, a 552 nm dichroic and a 560 nm long-pass filter (we chose long-pass emission filters that covered the full emission wavelength range, because Mac is a dim fluorophore and hardly contributed to the fluorescence emissions). For Arclight, we used the 480 nm LED from the Heliophore with a 470/30 nm excitation filter, a 498 nm dichroic mirror and a 500 nm long-pass emission filter. For in vivo imaging experiments with MacQ-mCitrine, we replaced the long-pass emission filter with a 534/30 nm emission filter. Illumination intensity in all cases was 15–30 mW mm −2 at the specimen plane. For imaging Mac’s native fluorescence, we used a 633 nm HeNe laser, a 632/22 nm excitation filter, a quad band 405/488/561/635 dichroic mirror and a 657 nm long-pass filter. We performed all Mac fluorescence imaging studies using 1,400 mW mm −2 illumination intensity at the specimen plane, due to its very weak fluorescence emission. An Andor iXon 897 electron-multiplying charge-coupled device camera cooled to –70 °C recorded the emission at 100–440 Hz, using binned pixels of 3 μm × 3 μm (or larger) in the image plane to achieve the image-acquisition speed. Alternatively, a Thorlabs PMM02 photomultiplier tube was used to take faster single cell optical traces (5 kHz) to determine kinetics. Cranial window for in vivo cerebellar imaging With the mice under isoflurane anaesthesia (1.5–2%), we first implanted a head plate over the cerebellum, opened a 3–4 mm diameter cranial window and removed the dura to expose the vermis of lobule V. To the exposed brain surface we applied artificial cerebrospinal fluid (ACSF: 125 mM NaCl, 5 mM KCl, 10 mM d -Glucose, 10 mM HEPES, 2 mM MgSO 4 , 2 mM CaCl 2 , pH 7.4). We stabilized the tissue using a glass cover slip secured with Kwik-Sil silicone elastomer and a retaining ring. For pharmacological studies, we re-exposed the tissue and applied CdCl 2 (10 μM in ACSF) for 10 min and then resealed the preparation to resume imaging. Computation of Δ F/F maps and time traces We computed maps of Δ F/F as the difference between the two images representing each pixel’s mean fluorescence intensity with and without the applied voltage step. Based on these maps, we ranked pixels according to their SNR, defined as , where is a pixel’s mean baseline fluorescence emission rate. To determine fluorescence time traces for individual cells, we aggregated the pixels that ranked in the top 20% of the SNR values. This subset of pixels sufficed to cover the cell soma. For the comparison of the steady-state SNR in Supplementary Fig. 3 , we defined a similar SNR as the one used for individual pixels, . Here, F norm is the mean fluorescence from each sensor collected from the selected pixels at the start of the imaging trace normalized to the starting intensity of the MacQ-mCitrine sensor, which had the highest brightness of the tested sensors. To compare the different sensors’ photon emission rates on an equal footing, we corrected for differences in illumination intensity and collection efficiency across experimental sessions. Determination of spike detection fidelity We defined the SNR for spike detection in a shot-noise limited optical trace ( Supplementary Fig. 4 ) as the peak value of in response to a spike, where F 0 is a neuron’s mean photon emission rate and ν is the sampling rate. This SNR is the peak response, Δ F , divided by the s.d. of the baseline, . We also computed iso-contours of SNR using this relation. In addition, we used a signal detection framework [29] to compute the spike discriminability parameter, d′ ( Figs 5d and 6d ). This parameter characterizes a sensor’s spike detection fidelity in a way that considers both the duration and the intensity of the fluorescence signal in response to action potentials. For studies in cultured neurons or in brain slices, we used experimental determinations of the mean baseline fluorescence intensity and the average fluorescence waveform in response to single action potentials (for example, Fig. 5c ) to compute d′ . This allowed us to make meaningful comparisons between sensors excited by different light sources with slightly different time variations in illumination intensity; by estimating the photon shot noise as the square root of the mean baseline fluorescence, rather than as its s.d., our calculation was more robust to light source intensity variations. We then computed iso-contours of d′ by approximating the fluorescence transients as mono-exponential decays, and computing the initial value of d′ from Δ F/F and the estimated total number of photons within the transient [29] . By comparison, for in vivo experiments we estimated d′ values based on the experimentally determined fluctuations in baseline fluorescence. Our reasoning behind this choice was that for in vivo experiments, fluctuations in fluorescence signals due to non-stationary factors such as brain motion and microcirculation are indelible aspects of brain imaging in live animals, and must be accounted for to provide realistic d′ values. Modelling fluorescence response to voltage transients We fit the kinetics in response to positive (depolarizing) membrane voltage transients (denoted with ‘+’) of the various sensors to the bi-exponential model: where A + is the normalizing amplitude, P +,fast is the percentage of the amplitude associated with the fast component, and τ +;{fast,slow} are the fast and slow time constants, respectively. We fit the kinetics in response to negative (hyperpolarizing) membrane voltage transients (denoted with ‘–’) of the various sensors to similar bi-exponential dynamics with a different set of coefficients, A – , P –,fast and τ –;{fast,slow} : We measured the probe optical response to an approximate +100 mV depolarization for 1 s for these fits. The model underlying our predicted frequency response and optical waveform response assumed that at steady-state conditions the difference of the fluorescence from baseline (Δ F ( t )= F ( t )— F 0 ) is proportional to the voltage depolarization: Δ F ( t )= AV m *( t ), where V m *( t )= V m ( t )— V 0 , where A is a proportionality constant, and F 0 is the fluorescence intensity at resting or holding voltage V 0 . However, outside steady-state the fluorescence reports a voltage, Δ F ( t )= AV * ( t )= A ( V ( t )— V 0 ), which differs from V m *( t ) due to the time lag that arises from the finite kinetics of the sensor’s response. Consistent with prior work on Arclight and rhodopsin based voltage sensors [17] , [28] , we found that the time-varying responses of both Arclight and MacQ-mCitrine well fit the double-exponential kinetics from above with a pair of time constants, τ fast and τ slow . Our model used the τ fast and τ slow as each having two different values depending on whether V m *( t )> V *( t ) or V m *( t )< V *( t ), matching the instantaneous on or off kinetics. Thus, when V m *( t )> V *( t ), we modelled the dynamics of the fluorescence intensity using the difference equation with the on kinetics: Similarly, when V m *( t )< V *( t ): Here τ {+,–};{fast,slow} and P {+,–};fast are defined in the same manner as defined in the kinetics measurements. Through these steps we determined the frequency response curve by computing the mean fluorescence response to a sinusoidally oscillating voltage, as a function of the oscillation frequency. We normalized the frequency response curves such that the response to a DC input matched the measured SNR of Supplementary Fig. 3 . Data and statistical analyses We used Matlab (Mathworks) to conduct all analyses. How to cite this article: Gong, Y. et al. Imaging neural spiking in brain tissue using FRET-opsin protein voltage sensors. Nat. Commun. 5:3674 doi: 10.1038/ncomms4674 (2014).